Two-dimensional vanadyl phosphate ultrathin nanosheets for high energy density and flexible pseudocapacitors Two-dimensional materials have been an ideal material platform for constructing flexible ultrathin-film supercapacitors, offering great advantages of flexibility, ultra-thinness and even transparency. Exploring new two-dimensional pseudocapacitive materials with high electrochemical activity is needed to achieve flexible ultrathin-film supercapacitors with higher energy densities. Here we report an inorganic graphene analogue, α 1 -vanadyl phosphate ultrathin nanosheets with less than six atomic layers, as a promising material to construct a flexible ultrathin-film pseudocapacitor in all-solid-state. The material exhibits a high potential plateau of ~ 1.0 V in aqueous solutions, approaching the electrochemical potential window of water (1.23 V). The as-established flexible supercapacitor achieves a high redox potential (1.0 V) and a high areal capacitance of 8,360.5 μF cm −2 , leading to a high energy density of 1.7 mWh cm −2 and a power density of 5.2 mW cm −2 . A rapidly growing demand for portable consumer electronics, such as flexible displays, mobile phones and notebook computers, has greatly promoted the development of flexible energy devices in all-solid-state [1] , [2] , [3] , [4] , [5] , [6] , [7] . As the future-generation energy storage device, the flexible thin-film supercapacitor in all-solid-state offers the synergic benefits of flexibility, thinness and transparency [2] , [8] , [9] , [10] , [11] , [12] . Among the different types of supercapacitors, pseudocapacitors have the advantage of a highly electroactive surface of the electrode materials owing to fast redox reaction, and exhibit much higher energy density compared with electrical double-layer capacitors as well as higher power density compared with lithium-ion batteries [13] , [14] , holding great promise for realizing high-performance flexible ultrathin-film supercapacitor in all-solid-state (FUSA) with pseudocapacitive behaviour [15] , [16] , [17] . Pursuing two-dimensional (2D) graphene-like materials with pseudocapacitive characteristics represents a promising direction to accomplish the flexible ultrathin-film pseudocapacitor in all-solid-state (FUPA) with higher energy density, and potentially excellent mechanical flexibility [18] , [19] , [20] . Moreover, obtaining the graphene-like pseudocapacitive materials not only requires the intrinsic layered structures that can be exfoliated into 2D ultrathin nanosheets, but also needs to possess a high electrochemical activity and high redox potential that can lead to higher energy density (E~ V 2 ). However, the development of graphene-like pseudocapacitive materials is still at its early stage, especially for the FUPAs with high power and energy densities. For example, the reversible redox Faradaic reactions occurred on the surface of layered Ni(OH) 2 and Co 3 O 4 exhibit the potential windows of only about 0.5 and 0.4 V, respectively [13] , [20] , both of which are still much lower than the limited electrochemical window of the aqueous solution (1.23 V) [21] . Therefore, the discovery of new graphene-like pseudocapacitive materials with enhanced electrochemical performance is much needed for constructing FUSA with higher power and energy densities, vital for satisfying the practical applications. Vanadyl phosphate (VOPO 4 ) has seen tremendous advances for layered materials with higher electrochemical performance [22] , [23] , [24] . Due to the enhanced inionicity of (V–O) bonds when (PO 4 ) 3− anion is introduced, V 4+ /V 5+ redox couple of VOPO 4 possesses the higher potential than that for simple vanadium oxide [25] . Layered VOPO 4 has a high redox potential of 1.0 V versus normal hydrogen electrode (NHE), and thus it is promising to establish the pseudocapacitors with improved energy density ( Supplementary Fig. S1 ) [26] , [27] . Furthermore, dehydrated vanadyl phosphate (VOPO 4 2H 2 O) has the characteristic layered structure, in which the sheets of VOPO 4 form from vertex-sharing VO 6 octahedra linking to phosphate PO 4 tetrahedra. Between each VOPO 4 layer, one water molecule coordinates with a vanadium atom through an oxygen atom and the other links adjacent layers together through weak hydrogen bonds ( Supplementary Fig. S2 ) [28] . The presence of weak hydrogen bonds in VOPO 4 ·2H 2 O provides the feasible clue to the exfoliation of layered VOPO 4 ·2H 2 O into VOPO 4 ultrathin nanosheets while maintaining the integrity of the in-plane structure. With the synergic advantages of high redox potential and the layered structure, the exfoliated VOPO 4 ultrathin nanosheets could be a promising new 2D graphene-like material with greatly enhanced electrochemical properties. Although VOPO 4 shows great potential for applications in flexible supercapacitors, its graphene-like material has long been unexplored in the past years, let alone the realization of the corresponding energy storage devices. Here we report a simple 2-propanol-assisted ultrasonication method to effectively exfoliate bulk VOPO 4 ·2H 2 O into VOPO 4 ultrathin nanosheets, with a thickness of less than six atomic layers, as a new graphene-like material. To fully explore the electrochemical performance of VOPO 4 , a VOPO 4 /graphene hybrid film was layer-by-layer assembled to achieve both high planar conductivity and superior electrochemical performance. The FUPA based on the VOPO 4 /graphene hybrid thin film demonstrated a high output voltage, a large specific capacitance and a high energy density, opening up opportunities for exploring new quasi-2D materials for flexible energy device with higher energy density. VOPO 4 ultrathin nanosheet The VOPO 4 ultrathin nanosheets were achieved by exfoliation of bulk VOPO 4 ·2H 2 O through a simple ultrasonication method in 2-propanol with a short reaction time of 15 min. For bulk VOPO 4 ·2H 2 O, VOPO 4 layers are linked together by hydrogen bonds from the interaction between H 2 O molecular and VOPO 4 layers. As one kind of weak intermolecular force, hydrogen bond is very sensitive to the applied external force [29] . For example, the applied strong ultrasonication provides the powerful force to trigger the breaking of hydrogen bonds. In our case, the exfoliation process from bulk VOPO 4 2H 2 O to VOPO 4 graphene-like material was conducted in 2-propanol solution, in that 2-propanol as a secondary alcohol is more suitable than primary alcohols as the dispersant due to the lower reactivity of hydroxyl group with the VOPO 4 layer matrix ( Supplementary Fig. S3 ). The interaction force of hydrogen bonds between 2-propanol and H 2 O further promoted the H 2 O molecules extracted from the interlayer space of bulk VOPO 4 ·2H 2 O. ( Fig. 1a ). The obtained VOPO 4 ultrathin nanosheets were homogeneously dispersed in solution with high stability for over several months. 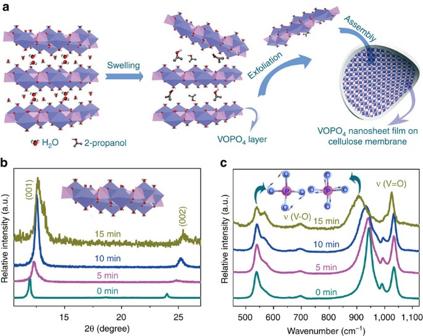Figure 1: Formation of VOPO4ultrathin nanosheets. (a) Schematic illustration for 2-propanol-assisted exfoliation process from bulk VOPO4·2H2O to graphene-like VOPO4nanosheets. During the process of ultrasonication in 2-propanol solution, the VOPO4layers were swelled and interlayered H2O molecules effused, resulting in the VOPO4ultrathin nanosheets. (b,c) XRD and Raman spectra of samples for the elongated ultrasonication time of 0, 5, 10 and 15 min, respectively. The insets incare the symmetric bending (left) and stretching (right) modes of O–P–O, respectively. Figure 1: Formation of VOPO 4 ultrathin nanosheets. ( a ) Schematic illustration for 2-propanol-assisted exfoliation process from bulk VOPO 4 ·2H 2 O to graphene-like VOPO 4 nanosheets. During the process of ultrasonication in 2-propanol solution, the VOPO 4 layers were swelled and interlayered H 2 O molecules effused, resulting in the VOPO 4 ultrathin nanosheets. ( b , c ) XRD and Raman spectra of samples for the elongated ultrasonication time of 0, 5, 10 and 15 min, respectively. The insets in c are the symmetric bending (left) and stretching (right) modes of O–P–O, respectively. Full size image The structural transformation process during the exfoliation could be revealed by the characterizations of X-ray powder diffraction (XRD) patterns and Raman spectra, which performed on the transferrable VOPO 4 thin films. The XRD characterization of vacuum-filtration assembled films of samples at different sonication time is shown in Fig. 1b . The XRD pattern at the initial sonication process can be readily indexed into the tetragonal VOPO 4 ·2H 2 O with the standard JCPDS card No.84-0111 (VOPO 4 ·2H 2 O, space group P4/nmm, a =6.202 Å, b =6.202 Å, c =7.410 Å). As the strong ultrasonication proceeds, the (001) peak became relatively stronger compared with other XRD peaks, revealing that the applied sonication waves triggered the structural arrangements and enhanced the c axis orientation for the formation process of high-quality 2D nanosheets. Furthermore, the (001) peak of VOPO 4 ·2H 2 O gradually shifted from lower 2θ (11.74°) to a higher one (13.5°) during the sonication process, indicating the decrease of the interlayer spacing distance from VOPO 4 ·2H 2 O to the final VOPO 4 ultrathin nanosheets as a result of the escape of molecular H 2 O from VOPO 4 interlayers. In addition, Raman spectra shown in Fig. 1c further verified structural evolutions during the exfoliation process. The bands at 937 cm −1 were assigned to the symmetric O–P–O stretching modes [30] , [31] . With the elongated exfoliation time, the red shift of Raman peaks of O–P–O stretching mode was more noticeable. Obviously, there was a strong microstructural correlation between symmetry of O–P–O stretching modes with the hydrogen bonding among the interlayered H 2 O molecular. With the breaking of hydrogen bonds from the oxygen atoms of the P–O bond in VOPO 4 , the mitigation of the steric hindrance would facilitate the occurrence of the O–P–O stretching modes with lower energy. However, the peaks related to the symmetric bending vibrations of O–P–O, V–O and V=O stretching mode demonstrated little shift with no obvious peak position evolution ( Supplementary Fig. S4 ). The Raman results confirmed that the exfoliated VOPO 4 nanosheets maintained the integrity of the in-plane VOPO 4 structure without obvious structural deformations. To unravel the microscopic outlook and structural crystallinity of exfoliated 2D VOPO 4 nanosheets, microstructural characterizations were performed. Scanning electron microscopy (SEM) images of the precursor VOPO 4 ·2H 2 O and graphene-like VOPO 4 nanosheets were taken and compared as shown in Fig. 2 and Supplementary Fig. S5 . The bulk VOPO 4 ·2H 2 O exhibited the typical layered structure, of which the layers were tightly stacked. In contrast, SEM image of the exfoliated products after 15 min ultransonication ( Fig. 2b ) shows the morphology of ultrathin nanosheets with a typical size ranging from 400 nm to several micrometres. Transmission electron microscopy (TEM) image of the exfoliated VOPO 4 nanosheet in Fig. 2c reveals a free-standing, sheet-like morphology with a lateral size of ~ 1 μm, and the nearly transparent feature implies the ultrathin thickness of exfoliated nanosheets. Atomic force microscopy image in Fig. 2d was taken to further evaluate the thickness of the VOPO 4 nanosheet. The measured height was ~ 4.07 nm, denoting that the nanosheet was comprised of 5–6 single layers, given that the c parameter of the VOPO 4 ·2H 2 O is 7.410 Å. The corresponding HR-TEM image and fast Fourier transform pattern are shown in Fig. 2e , demonstrating that the exfoliated sheets were single crystalline with [001] preferential orientation. The interplanar distance of 0.31 nm fits well with the plane distance of d 200 and d 202 , respectively. The orientation angle values 90° of these two planes of (200) and (020) in HR-TEM image and fast Fourier transform pattern was consistent with those calculated from tetragonal crystallographic parameters of VOPO 4 ·2H 2 O. These characterization results showed that VOPO 4 ·2H 2 O was successfully exfoliated into ultrathin VOPO 4 nanosheets that exhibited good crystallinity and high c axis orientation, providing strong basis for further assembly of VOPO 4 nanosheets into large-area practical energy storage devices. 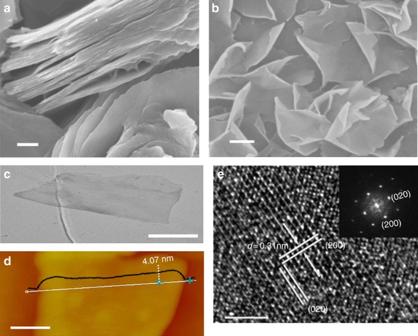Figure 2: Microstructural characterization of ultrathin nanosheets. (a) Field emission scanning electron microscopy image of bulk VOPO4·2H2O precursors, where the stacked layers can be clearly seen. Scale bar, 200 nm. (b) The SEM image of exfoliated VOPO4ultrathin nanosheets with warped edges exhibiting the ultrathin features. Scale bar, 200 nm. (c) TEM image of a typical ultrathin nanosheet. Scale bar, 500 nm. (d) Atomic force microscopy image of a typical nanosheet with a thickness of 4.07 nm, corresponding to less than six atomic layers. Scale bar, 100 nm. (e) High-resolution TEM (HR-TEM) image of a typical nanosheets showing the lattice fringes of (200) and (020) planes, and the inset is the corresponding fast Fourier transform patterns of the same area in the HR-TEM image. Scale bar, 2 nm. Figure 2: Microstructural characterization of ultrathin nanosheets. ( a ) Field emission scanning electron microscopy image of bulk VOPO 4 ·2H 2 O precursors, where the stacked layers can be clearly seen. Scale bar, 200 nm. ( b ) The SEM image of exfoliated VOPO 4 ultrathin nanosheets with warped edges exhibiting the ultrathin features. Scale bar, 200 nm. ( c ) TEM image of a typical ultrathin nanosheet. Scale bar, 500 nm. ( d ) Atomic force microscopy image of a typical nanosheet with a thickness of 4.07 nm, corresponding to less than six atomic layers. Scale bar, 100 nm. ( e ) High-resolution TEM (HR-TEM) image of a typical nanosheets showing the lattice fringes of (200) and (020) planes, and the inset is the corresponding fast Fourier transform patterns of the same area in the HR-TEM image. Scale bar, 2 nm. Full size image 2D hybrid thin film The bulk VOPO 4 is well known as a high-performance electrochemical material with a high redox voltage under aqueous solution of 1.0 V versus NHE, approaching the electrochemical window of water (1.23 V) [21] , which entails the great fascination for the construction of high-efficiency energy storage devices. ( Supplementary Fig. S1 ) In our work, VOPO 4 ultrathin nanosheets with <6 atomic layers, as a new inorganic graphene-like material, provide an ideal 2D material platform to investigate their electrochemical behaviour, and to give the feasibility to construct the FUPA. Because of the poor conductivity of VOPO 4 nanosheet, a layer-by-layer strategy was adopted to assemble a VOPO 4 /graphene hybrid film, and the hybrid thin film exhibits advantageous features of being uniform, compact and nearly transparent ( Fig. 3a ). The hybrid film could be readily transferred and free-standing due to its high-quality film structure. Fig. 3b is the cross-section SEM image of the hybrid film, showing the compact layer-by-layer structure with the thickness of ~ 90 nm thick. The inset in Fig. 3c is the SEM image of the smooth hybrid film, where the graphene was underneath VOPO 4 layers as illustrated by the white arrows. The combined analyses of the TEM and XRD results further reveal that the as-formed VOPO 4 /graphene hybrid film was the stacking of serial layers of chemically integrated VOPO 4 nanosheets on graphene sheets exhibiting the highly c axis crystalline orientation, in which the VOPO 4 nanosheets integrated on the graphene sheet as the building units and they assembled in stacks to form the final VOPO 4 /graphene hybrid films ( Supplementary Figs S6 and S7 ). To better understand the layer-by-layer assembly of VOPO 4 nanosheets with graphene, Fig. 3c shows the Raman spectra of VOPO 4 film, graphene film and VOPO 4 /graphene hybrid film, respectively. The brown line is the Raman spectrum of graphene, which possesses two pronounced peaks at 1,580 cm −1 (G) and 2,700 cm −1 (2D) of graphene. The stronger intensity of G peak shows that the synthesized graphene is of good quality and high crystallinity and the weaker D peak at ~ 1,347 cm −1 corresponds to the lower disordering [32] , [33] , [34] . The red line represents the Raman spectrum of VOPO 4 nanosheets film with characteristic peaks of VOPO 4 at ~ 866 cm −1 and 1,019 cm −1 corresponding to the symmetric stretching vibration ν 1 (PO 4 ) and V=O stretching mode. The Raman spectrum of VOPO 4 /graphene hybrid film (blue line) in Fig. 3c had the characteristic peaks of both VOPO 4 nanosheets and graphene with homogeneous distribution. The VOPO 4 /graphene hybrid films were of high-quality with uniform, compact, free-standing and high transparency features. 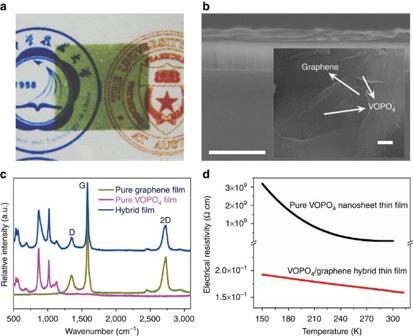Figure 3: Hybrid thin film of 2D VOPO4and graphene. (a) Demonstration of VOPO4/graphene hybrid thin film on the surface of PET substrate, exhibiting transparent feature. (b) The cross-section SEM image of the hybrid thin film with the thickness of ~ 90 nm. The surface of the hybrid film, of which the graphene lies under the VOPO4layers as indicated by the white arrows, is shown in the inset. Scale bar, 500 nm; Inset scale bar, 100 nm. (c) The Raman spectra of graphene film (brown line), VOPO4film (red line) and VOPO4/graphene hybrid film (blue line), respectively. (d) The temperature dependence of planar resistivity of the VOPO4/graphene hybrid film and pure VOPO4nanosheet thin film, where the incorporation of graphene greatly enhanced the electrical conductivity in the VOPO4/graphene hybrid film. Figure 3: Hybrid thin film of 2D VOPO 4 and graphene. ( a ) Demonstration of VOPO 4 /graphene hybrid thin film on the surface of PET substrate, exhibiting transparent feature. ( b ) The cross-section SEM image of the hybrid thin film with the thickness of ~ 90 nm. The surface of the hybrid film, of which the graphene lies under the VOPO 4 layers as indicated by the white arrows, is shown in the inset. Scale bar, 500 nm; Inset scale bar, 100 nm. ( c ) The Raman spectra of graphene film (brown line), VOPO 4 film (red line) and VOPO 4 /graphene hybrid film (blue line), respectively. ( d ) The temperature dependence of planar resistivity of the VOPO 4 /graphene hybrid film and pure VOPO 4 nanosheet thin film, where the incorporation of graphene greatly enhanced the electrical conductivity in the VOPO 4 /graphene hybrid film. Full size image In addition, hybrid VOPO 4 /graphene films exhibited greatly enhanced electrical properties. The hybrid film can be transferred onto various target substrates ( Supplementary Fig. S8 ) for electrical measurements. Temperature dependence of planar electrical resistivity of the VOPO 4 /graphene hybrid film was carried out as shown in Fig. 3d . As can be seen, the hybrid film possessed good conductivity in a wide temperature range from 150 to 300 K with slight resistivity change from 1.9 × 10 −1 Ω cm (150 K) to 1.6 × 10 −1 Ω cm (300 K), which is eight orders of magnitude lower than that of pure VOPO 4 nanosheet thin film (3.0 × 10 7 Ω cm at 300 K). With the VOPO 4 nanosheets integrated on the graphene layers, the 2D VOPO 4 /graphene hybrid film possessed the much improved electrical conductivity, making possible embodiment of outstanding electrochemical performance of VOPO 4 nanosheets. FUPA performance To further study the electrochemical properties of the VOPO 4 graphene-like materials, a FUPA based on 2D VOPO 4 /graphene hybrid film was fabricated. The FUPA devices were configured and fabricated according to the typical principles of flexiblity, ultra-thinness and all-solid-state, as illustrated in Fig. 4a . In this regard, VOPO 4 /graphene hybrid film was transferred onto the gold-coated polyethylene terephthalate (PET) sheet as the working electrode. The polyvinyl alcohol (PVA)/LiCl was introduced as the solid electrolyte and separator to prevent potential dissolving of active material of VOPO 4 nanosheets. Note that the salt LiCl could not be easily crystallized out during the process of gel drying and could provide a neutral pH medium, which makes PVA/LiCl an excellent electrolyte for vanadium-involved solid-state pseudocapacitors [35] . The as-assembled FUPA exhibited excellent electrochemical performance. 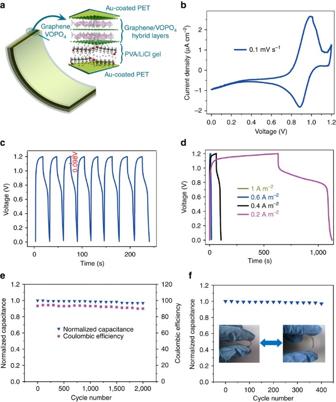Figure 4: Electrochemical performance. (a) Schematic illustration of an as-fabricated flexible ultrathin-film pseudocapacitor, in which the VOPO4/graphene hybrid layers function as the working electrode and PVA/LiCl gel functions as the electrolyte. (b) CV curves of VOPO4/graphene hybrid film in PVA/LiCl electrolyte from 0 to 1.2 V at 0.1 mV s−1. (c) Galvanostatic cycling behaviour of the as-fabricated FUPA and its IR drop. (d) Galvanostatic charge–discharge curves at different current density of 0.2, 0.4, 0.6 and 1 A m−2. (e) Cycle test of the VOPO4/graphene hybrid film-based FUPA over 2,000 cycles. (f) Cycling stability of the FUPA under repeated bending/extending deformation. Figure 4 summarizes the electrochemical performances of the as-fabricated FUPA based on VOPO 4 /graphene utrathin film with a thickness of ~ 90 nm. Figure 4b shows the cyclic voltammetry (CV) curve in the PVA/LiCl electrolyte from 0 to 1.2 V at scan rate of 0.1 mV s −1 . The obvious redox current peaks at ~ 1.1 V (oxidation peak) and 0.9 V (reduction peak) in the CV plots correspond to the reversible pseudocapacitive reactions of VOPO 4 nanosheets with Li + , which can be represented by the following equation: Figure 4: Electrochemical performance. ( a ) Schematic illustration of an as-fabricated flexible ultrathin-film pseudocapacitor, in which the VOPO 4 /graphene hybrid layers function as the working electrode and PVA/LiCl gel functions as the electrolyte. ( b ) CV curves of VOPO 4 /graphene hybrid film in PVA/LiCl electrolyte from 0 to 1.2 V at 0.1 mV s −1 . ( c ) Galvanostatic cycling behaviour of the as-fabricated FUPA and its IR drop. ( d ) Galvanostatic charge–discharge curves at different current density of 0.2, 0.4, 0.6 and 1 A m −2 . ( e ) Cycle test of the VOPO 4 /graphene hybrid film-based FUPA over 2,000 cycles. ( f ) Cycling stability of the FUPA under repeated bending/extending deformation. Full size image The slight internal resistance (IR) drop of 0.098 V observed in Fig. 4c implied a small intrinsic series resistance of VOPO 4 /graphene hybrid film. Figure 4c shows the galvanostatic charge–discharge curves of the VOPO 4 /graphene-based FUPA, from which the specific capacitance is calculated to be 8,360.5 μF cm −2 at current density of 0.2 A m −2 ( Supplementary Tables S1 and S2 ). Our areal capacitance of 8,360.5 μF cm −2 (that is, 928.9 F cm −3 ) is the highest value among all reported FUSAs [18] , [19] , [20] , [36] . The electrochemical performance of 2D VOPO 4 /graphene hybrid thin film is superior to that of bulk VOPO 4 , that of pure 2D VOPO 4 nanosheets and even to that of other crystal forms of VOPO 4 . ( Supplementary Figs S9—S12 ). Moreover, the FUPAs fabricated with higher mass loading of active materials (thickness up to ~ 10 μm) can still maintain good electrochemical performance, in which the areal capacitance increased 72 times when the thickness of electrode increased from ~ 90 nm to ~ 10 μm. ( Supplementary Fig. S13 ). Employing pseudocapacitor in-plane, micro-electrodes can potentially further enhance the performance of 2D hybrid VOPO4/graphene thin film, as it could mitigate the issues from contact resistance and electrolyte ions diffusion in the case of much higher mass loading [10] , [37] . Furthermore, the discharge voltage up to ~ 1.0 V is a significant step for constructing high energy density supercapacitors. Our reported discharge voltage up to 1.0 V is a fairly high value compared with previously reported supercapacitors in the aqueous electrolytes [13] , [14] , [15] , [16] , [17] , [18] , [19] , [20] . The high specific capacitance (8,360.5 μF cm −2 ) and redox voltage (up to 1.0 V) lead to the ultrahigh energy density of 1.7 mWh cm −2 and power density of 5.2 mW cm −2 . These are the highest values among the reported FUSAs as shown in Fig. 5 ( Supplementary Tables S1 and S2 ). The improved energy density of FUSA with its high power density would make it more competitive for practical applications of energy storage devices [38] . 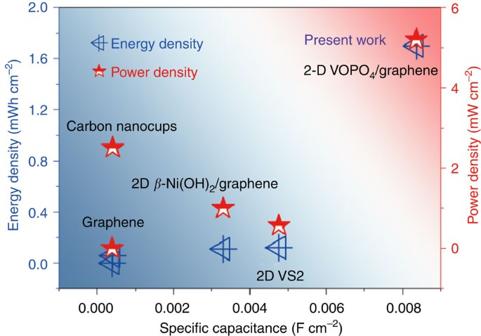Figure 5: Performance comparison of various materials. Our FUPA based on 2D VOPO4/graphene hybrid thin film showing the best performance of energy density compared with the reported flexible ultrathin-film supercapacitors in all-solid-state for graphene18, carbon nanocups36, Ni(OH)2(ref.20) and 2D VS2(ref.19). Figure 5: Performance comparison of various materials. Our FUPA based on 2D VOPO 4 /graphene hybrid thin film showing the best performance of energy density compared with the reported flexible ultrathin-film supercapacitors in all-solid-state for graphene [18] , carbon nanocups [36] , Ni(OH) 2 (ref. 20 ) and 2D VS 2 (ref. 19 ). Full size image As shown in Fig. 4e , the as-fabricated FUPA had an excellent cycle life, as after 2,000 charge–discharge cycles specific capacitance retained 96% of the initial capacitance and Columbic efficiency was kept at ~ 90%, demonstrating excellent long-term cycling stability. Figure 4f demonstrates the excellent flexibility of the as-fabricated FUPA with negligible degradation of the specific capacitance even after 400 bending cycles. In short, the graphene-like VOPO 4 materials have shown the fascinating electrochemical and mechnical characteristics for practical applications in high-performance, flexible energy storage devices catering for portable and flexible electronics. In summary, VOPO 4 ultrathin nanosheets with less than six atomic layers, as a new inorganic graphene-like material, have been reported for the first time. The as-fabricated FUPAs based on hybrid structure of the newly found VOPO 4 ultrathin nanosheets and graphene sheets exhibit extremely high specific capacitance (up to 8,360.5 μF cm −2 ), high redox voltage (up to 1 V), long cycle life (more than 2,000 cycles) and excellent flexibility, leading to an ultrahigh energy density of 1.7 mWh cm −2 and a power density of 5.2 mW cm −2 . Our findings represent a promising direction and a significant step towards exploring new quasi-2D materials for flexible energy device with higher energy density in the near future. Synthesis of bulk VOPO 4 ·2H 2 O Bulk VOPO 4 2H 2 O was obtained according to a simple method reported in the previous literature [39] . The mixture, including V 2 O 5 (4.8 g), H 3 PO 4 (85% 26.6 ml) and H 2 O (115.4 ml), was refluxed at 110 °C for 16 h. Thereafter, the system was permitted cool down to room temperature. The yellow precipitate was finally collected by filtration and washed several times with water and acetone. The resulting sample was dried in vacuum at 60 °C for 3 h. Assembly of the hybrid VOPO4/graphene film The graphene used in our experiments was synthesized according to the procedure used in previous studies [40] , [41] . The VOPO 4 /graphene hybrid film was assembled by a layer-by-layer strategy. Specifically, the VOPO 4 and graphene dispersion were vacuum filtered in turns over a cellulose membrane with 0.22 μm pore size to form a homogeneous thin film. The thickness of the hybrid thin film can be tuned by changing the filtrated amount of the VOPO 4 and graphene dispersion. Preparation of gel electrolyte Four grams of PVA powder was put into 40 ml distilled water with stirring at 95 °C (ref. 35 ). When the PVA powder was completely dissolved, 8.5 g LiCl was added into the solution under vigorous stirring. After the LiCl/PVA turned to into a transparent and clear gel, it was cooled down at room temperature. At last, the LiCl gel electrolyte was prepared. Exfoliation of bulk precursor into graphene-like material Bulk VOPO 4 ·2H 2 O (30 mg) was dispersed in a sealed glass bottle with 25 ml 2-propanol and then the dispersion was ultrasonicated in iced water for 15 min forming the VOPO 4 ultrathin nanosheets. The resultant yellow suspension was collected by vacuum filtration with a 0.22-μm pore size cellulose membrane, forming a homogeneous thin film, which can be easily transferred to arbitrary substrates by pressing another side of the cellulose membrane. Fabrication of flexible supercapacitors in all-solid-state FUPA devices typically include the working electrode, counter electrode, current collector and the flexible substrate. VOPO 4 /graphene hybrid film was transferred onto the gold-coated PET sheet as the working electrode, in which the mass percentage of VOPO 4 in the electrodes was ~ 65% measured by inductively coupled plasma emission spectroscopy. The gold-coated PET sheet was used as the counter electrode; gold-coated PET sheet served dual functions as both the current collector and the flexible substrate. Meanwhile, PVA/LiCl was introduced as the solid electrolyte and separator to prevent the possible dissolving of the active material of VOPO 4 nanosheets. The whole device was sealed carefully by the common transparent tape to make sure the device system is at a stable state. Material characterizations XRD was performed on a Philips X, Pert Pro Super diffractometer with Cu Kα radiation ( λ =1.54178 Å). Raman spectra were recorded at room temperature with a LABRAM-HR confocal laser micro Raman spectrometer 750 K with a laser power of 0.5 mW. The TEM images were taken on a JEOL-2010 transmission electron microscope at an acceleration voltage of 200 kV. The field emission scanning electron microscopy images were obtained on a JEOL JSM-6700F SEM. High-resolution TEM images were taken on a JEOL-2010 microscope at an accelerating voltage of 200 kV. Tapping-mode atomic force microscopy images were taken on a DI Innova Multimode SPM platform. Electrochemical performance of the supercapacitor was studied in a two-electrode system by CV and galvanostatic charge–discharge at an electrochemical station (CHI660B). Potential range set for galvanostatic charge–discharge tests was from 0 to 1.2 V. How to cite this article: Wu, C. et al . Two-dimensional vanadyl phosphate ultrathin nanosheets for high energy density and flexible pseudocapacitors. Nat. Commun. 4:2431 doi: 10.1038/ncomms3431 (2013).